Bhlhe40 controls cytokine production by T cells and is essential for pathogenicity in autoimmune neuroinflammation T H 1 and T H 17 cells mediate neuroinflammation in experimental autoimmune encephalomyelitis (EAE), a mouse model of multiple sclerosis. Pathogenic T H cells in EAE must produce the pro-inflammatory cytokine granulocyte-macrophage colony stimulating factor (GM-CSF). T H cell pathogenicity in EAE is also regulated by cell-intrinsic production of the immunosuppressive cytokine interleukin 10 (IL-10). Here we demonstrate that mice deficient for the basic helix–loop–helix (bHLH) transcription factor Bhlhe40 ( Bhlhe40 −/− ) are resistant to the induction of EAE. Bhlhe40 is required in vivo in a T cell-intrinsic manner, where it positively regulates the production of GM-CSF and negatively regulates the production of IL-10. In vitro , GM-CSF secretion is selectively abrogated in polarized Bhlhe40 −/− T H 1 and T H 17 cells, and these cells show increased production of IL-10. Blockade of IL-10 receptor in Bhlhe40 −/− mice renders them susceptible to EAE. These findings identify Bhlhe40 as a critical regulator of autoreactive T-cell pathogenicity. Experimental autoimmune encephalomyelitis (EAE) serves as an animal model for the human neuroinflammatory disease multiple sclerosis. Encephalomyelitis in C57BL/6 mice in response to immunization with a peptide from myelin oligodendrocyte glycoprotein (MOG) is driven by cytokine-producing autoreactive T helper (T H ) cells [1] . Historically, interferon-γ (IFN-γ)-producing T H 1 cells were thought to be responsible for EAE, but recent evidence has revealed a more important role for interleukin 17 (IL-17)-producing T H 17 cells [2] , [3] . Nevertheless, neither T H 1 (IFN-γ) nor T H 17 (IL-17A, IL-17F, IL-21 and IL-22) signature cytokines are required for the development of EAE [4] , [5] , [6] , [7] . Instead, the cytokine granulocyte-macrophage colony stimulating factor (GM-CSF) has proven to be a critical factor in the encephalitogenicity of both T H 1 and T H 17 cells [8] , [9] , [10] , [11] , [12] . IL-1 receptor and IL-23 receptor signalling are required for T H cell production of GM-CSF during EAE [10] , [11] , [13] . GM-CSF production by T cells is regulated cell-intrinsically through the action of transcription factors. Factors that regulate its transcription include AP-1 family members, NFAT, NF-κB family members, including c-Rel and NF-κB1, and RUNX1 (refs 14 , 15 , 16 , 17 , 18 , 19 ). Recently, Codarri et al. [10] reported a requirement for RORγt for maximal production of GM-CSF by T H 17 cells, although a second report observed no reduction in GM-CSF secretion by Rorc −/− T H cells in vitro [11] . T H 1 cells also produce GM-CSF during EAE, yet specific transcription factors regulating their production of GM-CSF have not been identified [12] . Immunoregulatory cytokines, including IL-10, modulate the development of EAE [20] . IL-10 is produced by several cell types during EAE, including autoreactive non-pathogenic T H cells [21] , [22] , [23] , [24] , [25] , [26] , [27] . IL-10 suppresses effector T cell responses and limits inflammation. IL-10-deficient mice develop more severe EAE than wild-type (WT) mice [28] , [29] , [30] . Expression of IL-10 in T H cells can be regulated by several transcription factors, depending on the T H cell subset and the cytokine environment [31] , [32] , [33] , [34] , [35] . Relevant to EAE is the production of IL-10 by T H 1, T H 17, Tr1 cells and T regulatory cells (Tregs). Bhlhe40 (also known as Dec1, Stra13, Sharp2 or Bhlhb2) belongs to a family of basic helix–loop–helix transcriptional regulators sharing structural features including a basic DNA-binding domain, a helix–loop–helix domain mediating dimerization and a protein–protein interaction ‘Orange domain’ [36] , [37] . Members of this family are known to respond to environmental stimuli and regulate several physiological processes in diverse cell types, including the cell cycle, apoptosis and differentiation via their actions as both transcriptional activators and repressors. Bhlhe40 is expressed in T cells upon T-cell receptor (TCR) stimulation [38] . Bhlhe40 −/− mice develop a non-fully penetrant late-onset (age greater than ~8 months) lymphoproliferative disease associated with autoantibodies [38] , [39] , which may be due to a requirement for Bhlhe40 for Treg maintenance during ageing. Penetrance of this age-related disease appears to be influenced by genetic background. How Bhlhe40 regulates effector T-cell responses is incompletely characterized. In this study, we show that Bhlhe40 −/− mice are resistant to EAE induction due, at least in part, to a T H cell-intrinsic defect. T H cells from these mice display nearly normal IFN-γ and IL-17A production in T H 1 and T H 17 cultures, respectively, and produce these cytokines after immunization, but fail to mediate EAE. Instead, transcriptional and phenotypic analyses of Bhlhe40 −/− T H cells reveal that they fail to produce GM-CSF. We also demonstrate a role for Bhlhe40 in GM-CSF production by γδ T cells. Bhlhe40 −/− T H 1 and T H 17 cells produce increased amounts of IL-10, consistent with their nonencepahlitogenic phenotype. Moreover, blockade of IL-10 signalling renders Bhlhe40 −/− mice susceptible to EAE. Chromatin immunoprecipitation sequencing (ChIP-Seq) reveals binding of Bhlhe40 to the Il3 / Csf2 and Il10 loci at several sites bound by other transcriptional regulators. Overall, our results identify Bhlhe40 as a novel factor regulating GM-CSF and IL-10 production by T cells, and one that is required for autoimmune neuroinflammation. Bhlhe40-deficient mice are protected from EAE To examine the role of Bhlhe40 in autoimmunity, we immunized Bhlhe40 −/− mice with MOG peptide (amino acids 35–55 (MOG(35–55)). Bhlhe40 −/− mice were markedly resistant to EAE ( Fig. 1a ), showing no leukocyte infiltration on histological examination of spinal cord sections ( Fig. 1b ). Bhlhe40 was required by the hematopoietic compartment for EAE susceptibility, since reconstitution of irradiated Bhlhe40 −/− mice with WT bone marrow (BM) caused susceptibility to EAE, whereas reconstitution of WT mice with Bhlhe40 −/− BM engendered EAE resistance ( Fig. 1c ). Bhlhe40 is expressed in activated T H cell subsets ( Supplementary Fig. 1a ), as previously reported [38] , [40] . Transfer of WT and Bhlhe40 −/− T H cells each reconstituted the T-cell compartment of recipient Rag1 −/− mice equally ( Supplementary Fig. 1b ), but only WT cells, and not Bhlhe40 −/− cells, allowed development of EAE after immunization ( Fig. 1d ). 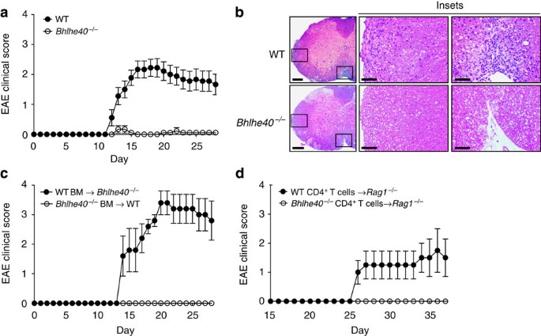Figure 1: Bhlhe40-deficient mice are protected from EAE. (a) Mean clinical scores of EAE in immunized WT (n=18) orBhlhe40−/−mice (n=18). Data are combined from four independent experiments. Incidence of disease: WT mice 17/18,Bhlhe40−/−mice 2/18. (b) H&E staining of spinal cord sections from WT andBhlhe40−/−mice at day 13 after EAE induction. Scale bars: 200 μm in left images, 50 μm in insets. (c) Mean clinical scores of EAE in BM chimeric mice 13 weeks after bone marrow reconstitution (n=5 per group). (d) Mean clinical scores of EAE inRag1−/−mice that received CD4+T cells from either WT orBhlhe40−/−mice 1 day before immunization (n=4 per group). For all figures throughout, error bars show mean±s.e.m. Figure 1: Bhlhe40-deficient mice are protected from EAE. ( a ) Mean clinical scores of EAE in immunized WT ( n =18) or Bhlhe40 −/− mice ( n =18). Data are combined from four independent experiments. Incidence of disease: WT mice 17/18, Bhlhe40 −/− mice 2/18. ( b ) H&E staining of spinal cord sections from WT and Bhlhe40 −/− mice at day 13 after EAE induction. Scale bars: 200 μm in left images, 50 μm in insets. ( c ) Mean clinical scores of EAE in BM chimeric mice 13 weeks after bone marrow reconstitution ( n =5 per group). ( d ) Mean clinical scores of EAE in Rag1 −/− mice that received CD4 + T cells from either WT or Bhlhe40 −/− mice 1 day before immunization ( n =4 per group). For all figures throughout, error bars show mean±s.e.m. Full size image The central nervous system (CNS) from MOG(35–55)-immunized Bhlhe40 −/− mice had reduced infiltrating myeloid cells (CD45 hi CD11b + ) relative to WT mice. In Bhlhe40 −/− mice, these cells lacked MHC class II expression, as did resident microglia (CD45 int CD11b + ) ( Fig. 2a,b ). Immunized Bhlhe40 −/− mice also harboured fewer CNS-infiltrating CD4 + T cells ( Fig. 2c ). CNS-infiltrating CD4 + T cells in WT mice produced IFN-γ and IL-17A, while the few CNS-infiltrating CD4 + T cells in Bhlhe40 −/− mice had reduced IFN-γ and IL-17A production ( Fig. 2d,e ). Notably, WT CD4 + T cells produced GM-CSF, but this was reduced by ~90% in Bhlhe40 −/− mice ( Fig. 2d,e and Supplementary Fig. 2a ). WT and Bhlhe40 −/− mice showed a similar low frequency of IL-10-producing CD4 + T cells in the CNS at the peak of disease ( Supplementary Fig. 2b ). Bhlhe40 −/− mice showed a slight reduction in the frequency of CNS-infiltrating Foxp3 + CD4 + T cells (analysed at day 29 after immunization, Supplementary Fig. 2c ). 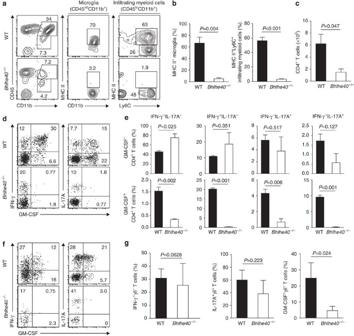Figure 2:Diminished neuroinflammation inBhlhe40−/−mice. (a) Flow cytometry of CNS myeloid cells from WT andBhlhe40−/−mice (n=3 per group) on day 16 after immunization. (b) Percentage of MHC class II+microglia and infiltrating myeloid cells. (c–e) Flow cytometry of CD4+T cells in the CNS of WT andBhlhe40−/−mice (n=3 per group) on day 16 after immunization. (c) CD4+T cell number. (d) Representative ICS for the indicated cytokines. (e) Frequency of CD4+T cells secreting each of the indicated eight possible combinations of GM-CSF, IL-17A and IFN-γ. (f,g) Flow cytometry of γδ T cells in the CNS of WT andBhlhe40−/−mice (n=3 per group) on day 14 after immunization. (f) Representative ICS for IFN-γ, IL-17A and GM- CSF. (g) Frequency of γδ T cells secreting IFN-γ, IL-17A or GM-CSF. Figure 2: Diminished neuroinflammation in Bhlhe40 −/− mice. ( a ) Flow cytometry of CNS myeloid cells from WT and Bhlhe40 −/− mice ( n =3 per group) on day 16 after immunization. ( b ) Percentage of MHC class II + microglia and infiltrating myeloid cells. ( c – e ) Flow cytometry of CD4 + T cells in the CNS of WT and Bhlhe40 −/− mice ( n =3 per group) on day 16 after immunization. ( c ) CD4 + T cell number. ( d ) Representative ICS for the indicated cytokines. ( e ) Frequency of CD4 + T cells secreting each of the indicated eight possible combinations of GM-CSF, IL-17A and IFN-γ. ( f , g ) Flow cytometry of γδ T cells in the CNS of WT and Bhlhe40 −/− mice ( n =3 per group) on day 14 after immunization. ( f ) Representative ICS for IFN-γ, IL-17A and GM- CSF. ( g ) Frequency of γδ T cells secreting IFN-γ, IL-17A or GM-CSF. Full size image γδ T cells are known to infiltrate the CNS during EAE, and promote neuroinflammation via their production of IL-17 and GM-CSF [13] , [41] . The role of IFN-γ production by these cells in this setting is unclear. Immunized Bhlhe40 −/− mice harboured ~30-fold fewer CNS-infiltrating γδ T cells compared with WT mice. Bhlhe40 −/− γδ T cells produced similar levels of IFN-γ and partially reduced levels of IL-17A, but more markedly reduced levels of GM-CSF ( Fig. 2f,g ). Together with our observations on significantly reduced GM-CSF production by Bhlhe40 −/− CD4 + T cells, these results suggest that Bhlhe40 is required for GM-CSF production by pathogenic T cells during neuroinflammation. We also tested an adoptive transfer EAE system in which a WT T H 1-polarized MOG(35–55)-specific T cell line was transferred to WT or Bhlhe40 −/− recipients [42] . These T cells produced IFN-γ and GM-CSF, but not IL-17A, upon stimulation ( Supplementary Fig. 2d ). When 5 million T cells were transferred, Bhlhe40 −/− mice were protected from EAE, although when 10 million T cells were transferred, Bhlhe40 −/− and WT mice both showed a similar incidence and severity of EAE ( Supplementary Fig. 2e,f ). We speculate that these results are the result of a requirement for Bhlhe40 in host T cells during the induction of neuroinflammation by low numbers of adoptively transferred MOG-specific T cells. Overall, our results indicate a role for Bhlhe40 in both immunization-induced and passive EAE. Bhlhe40 regulates T-cell cytokine production after immunization Draining lymph nodes (DLNs) from immunized Bhlhe40 −/− mice had reduced cellularity relative to WT mice ( Supplementary Fig. 3a ). Flow cytometry of these DLNs indicated normal frequencies of lymphoid and myeloid cell populations, indicating that the decreased cellularity was not due to the reduction in a particular cell type ( Supplementary Fig. 3b ). Similar frequencies of interleukin 2 (IL-2)- and IFN-γ-producing T cells and a modest reduction in the frequency of IL-17A-producing T cells were observed in DLNs from Bhlhe40 −/− mice relative to WT mice in response to stimulation with MOG(35–55) or concanavalin A (ConA) as measured by ELISPOT assays ( Fig. 3a ). Consistent with their decreased IL-17A production, the frequency of RORγt + CD4 + T cells was moderately decreased in DLNs of Bhlhe40 −/− mice ( Supplementary Fig. 4a,b ). DLNs from Bhlhe40 −/− mice showed a markedly reduced frequency of MOG(35–55)-specific GM-CSF-producing T cells relative to WT mice, and an increased frequency of MOG(35–55)-specific IL-10-producing T cells ( Fig. 3b ). Intracellular cytokine staining (ICS) of DLN cells also showed diminished GM-CSF ( Supplementary Fig. 4c,d ) and increased IL-10 production ( Supplementary Fig. 4e,f ) from Bhlhe40 −/− CD4 + T cells. The defect in GM-CSF production by Bhlhe40 −/− CD4 + T cells could not be fully restored in vitro by culture with IL-1β or IL-23, cytokines that are reported to promote GM-CSF secretion [10] , [11] , [12] , [13] ( Fig. 3c,d ). The increased IL-10 production by Bhlhe40 −/− CD4 + T cells was significantly augmented by in vitro culture with IL-12 ( Fig. 3e,f ). 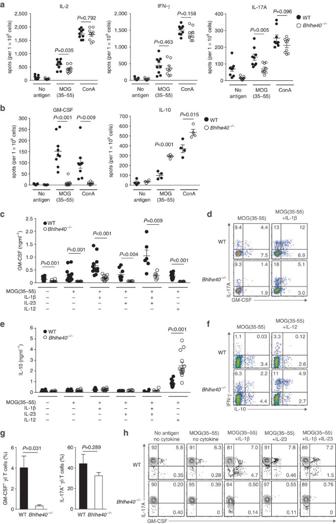Figure 3: T cells require Bhlhe40 for normal cytokine production after immunization. (a,b) ELISPOT assays for the quantitation of cells secreting (a) IL-2, IFN-γ, and IL-17A or (b) GM-CSF and IL-10 performed on DLN cells 7 days after immunization of WT andBhlhe40−/−mice. Data for IL-2, IFN-γ, IL-17A and GM-CSF are combined from three independent experiments (n=9 mice per group). Data for IL-10 is from one representative experiment of two (n=4 mice per group). (c,e) DLN cells from immunized WT andBhlhe40−/−mice (n=14 per group) were cultured with or without MOG(35–55) and with or without IL-1β, IL-23 and/or IL-12 as indicated. (c) GM-CSF or (e) IL-10 was measured in the supernatant at day 4. Data are combined from five independent experiments. Cells from all mice were not used in all conditions in each of the four experiments. (d) DLN cells from immunized WT andBhlhe40−/−mice were cultured with MOG(35–55) with or without IL-1β for 4 days, followed by ICS. Representative plots are gated on CD4+T cells. (f) DLN cells from immunized WT andBhlhe40−/−mice were cultured with MOG(35–55) with or without IL-12 for 4 days, followed by ICS. Representative plots are gated on CD4+T cells. (g) Frequencies of GM-CSF+and IL-17A+γδ T cells in DLNs 7 days after immunization of WT andBhlhe40−/−mice (n=3 per group) as determined by ICS. (h) DLN cells from immunized WT andBhlhe40−/−mice were cultured with or without MOG(35–55) and with or without IL-1β and/or IL-23 as indicated for 4 days. Cells were stimulated with PMA/ionomycin in the presence of brefeldin A for 4 h and then analysed for IL-17A and GM-CSF by intracellular staining (that is, our normal ICS protocol). Representative plots are gated on γδ T cells. Figure 3: T cells require Bhlhe40 for normal cytokine production after immunization. ( a , b ) ELISPOT assays for the quantitation of cells secreting ( a ) IL-2, IFN-γ, and IL-17A or ( b ) GM-CSF and IL-10 performed on DLN cells 7 days after immunization of WT and Bhlhe40 −/− mice. Data for IL-2, IFN-γ, IL-17A and GM-CSF are combined from three independent experiments ( n =9 mice per group). Data for IL-10 is from one representative experiment of two ( n =4 mice per group). ( c , e ) DLN cells from immunized WT and Bhlhe40 −/− mice ( n =14 per group) were cultured with or without MOG(35–55) and with or without IL-1β, IL-23 and/or IL-12 as indicated. ( c ) GM-CSF or ( e ) IL-10 was measured in the supernatant at day 4. Data are combined from five independent experiments. Cells from all mice were not used in all conditions in each of the four experiments. ( d ) DLN cells from immunized WT and Bhlhe40 −/− mice were cultured with MOG(35–55) with or without IL-1β for 4 days, followed by ICS. Representative plots are gated on CD4 + T cells. ( f ) DLN cells from immunized WT and Bhlhe40 −/− mice were cultured with MOG(35–55) with or without IL-12 for 4 days, followed by ICS. Representative plots are gated on CD4 + T cells. ( g ) Frequencies of GM-CSF + and IL-17A + γδ T cells in DLNs 7 days after immunization of WT and Bhlhe40 −/− mice ( n =3 per group) as determined by ICS. ( h ) DLN cells from immunized WT and Bhlhe40 −/− mice were cultured with or without MOG(35–55) and with or without IL-1β and/or IL-23 as indicated for 4 days. Cells were stimulated with PMA/ionomycin in the presence of brefeldin A for 4 h and then analysed for IL-17A and GM-CSF by intracellular staining (that is, our normal ICS protocol). Representative plots are gated on γδ T cells. Full size image We analysed cytokine production by Bhlhe40 −/− T cells in three additional settings. First, instead of using the self-peptide MOG(35–55), we immunized mice with the foreign, MHC class II-restricted peptide of chicken ovalbumin (OVA(323–339)). Again, Bhlhe40 −/− CD4 + T cells failed to produce GM-CSF following this immunization, with intact IL-2 and IFN-γ production, and partially decreased IL-17A production ( Supplementary Fig. 4g ). Second, we analysed CD4 + T-cell cytokine responses in immunized mixed BM chimeric mice. Bhlhe40 −/− T cells showed a T cell-intrinsic defect in GM-CSF secretion in this setting, with normal IL-17A secretion ( Supplementary Fig. 4h,i ). Third, we analysed cytokine responses in immunized Rag1 −/− mice that had received transfers of purified WT or Bhlhe40 −/− CD4 + T cells ( Supplementary Fig. 5 ). Bhlhe40 −/− CD4 + T cells showed reduced GM-CSF and increased IL-10 production in this setting, with normal IFN-γ production. For unclear reasons, IL-17A secretion by Bhlhe40 −/− CD4 + T cells appeared decreased in the spleen, but increased in the DLN in this setting. γδ T cells in the DLNs of immunized Bhlhe40 −/− mice also showed a selective loss of GM-CSF production that could not be restored by in vitro culture with IL-1β and/or IL-23 ( Fig. 3g,h ). Naive splenic γδ T cells from non-immunized Bhlhe40 −/− mice were capable of responding to IL-1β, IL-23 and IL-12 (refs 41 , 43 ), as demonstrated by their increased size and granularity, but failed to produce normal levels of GM-CSF in these cultures ( Supplementary Fig. 6a,b ). Overall, these results assessing T-cell responses in the periphery in combination with our findings in the CNS indicate that both CD4 + and γδ T cells require Bhlhe40 to produce GM-CSF. Bhlhe40 regulates cytokine production by in vitro polarized T H cells We tested whether Bhlhe40 −/− CD4 + T cells responded normally to in vitro activation. Stimulation with plate-bound anti-CD3 alone or anti-CD3 and anti-CD28 led to normal IL-2 secretion, reduced GM-CSF secretion and increased IL-10 secretion by Bhlhe40 −/− CD4 + T cells ( Supplementary Fig. 7a–c ). We next examined cytokine production by in vitro polarized T H cells from WT and Bhlhe40 −/− mice. In general, polarized T H cells from Bhlhe40 −/− mice showed normal production of their signature cytokines, although Bhlhe40 −/− T H 1 cells showed a ~40% decrease in IFN-γ production, consistent with a previous report [39] ( Fig. 4a,b ). Consistent with these cytokine results, we found decreased expression of the transcription factor T-bet in Bhlhe40 −/− T H 1 cells, with nearly normal expression of Gata-3 and RORγt in Bhlhe40 −/− T H 2 and T H 17 cells, respectively ( Supplementary Fig. 7e ). 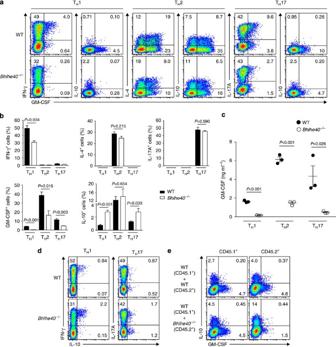Figure 4:THcells require Bhlhe40 for normal cytokine productionin vitro. (a–d) CD4+T cells from WT andBhlhe40−/−mice (n=3 per group) were polarized in TH1, TH2 or TH17 culture conditions for 4 days. (a) Representative ICS for the indicated cytokines. (b) Frequencies of IFN-γ+, IL-4+, IL-17A+, GM-CSF+and IL-10+cells in TH1, TH2 and TH17 cultures. (c) TH1, TH2 and TH17 cells were stimulated for 24 h with anti-CD3 and anti-CD28. GM-CSF was measured in the supernatant by ELISA. (d) Representative ICS for the indicated cytokines. (e) CD4+T cells from the indicated congenic mice were mixed prior to culturing in non-polarizing conditions for 4 days, followed by ICS. Cells were gated based on their expression of CD45.1 or CD45.2. Representative ICS for IL-10 and GM-CSF is shown. Figure 4: T H cells require Bhlhe40 for normal cytokine production in vitro . ( a – d ) CD4 + T cells from WT and Bhlhe40 −/− mice ( n =3 per group) were polarized in T H 1, T H 2 or T H 17 culture conditions for 4 days. ( a ) Representative ICS for the indicated cytokines. ( b ) Frequencies of IFN-γ + , IL-4 + , IL-17A + , GM-CSF + and IL-10 + cells in T H 1, T H 2 and T H 17 cultures. ( c ) T H 1, T H 2 and T H 17 cells were stimulated for 24 h with anti-CD3 and anti-CD28. GM-CSF was measured in the supernatant by ELISA. ( d ) Representative ICS for the indicated cytokines. ( e ) CD4 + T cells from the indicated congenic mice were mixed prior to culturing in non-polarizing conditions for 4 days, followed by ICS. Cells were gated based on their expression of CD45.1 or CD45.2. Representative ICS for IL-10 and GM-CSF is shown. Full size image GM-CSF production varied between WT T H 1, T H 2 and T H 17 cells, with the least production of GM-CSF found in T H 1 cultures ( Fig. 4a–c ), consistent with an earlier report [10] . Bhlhe40 −/− T cells showed markedly reduced production of GM-CSF under all conditions of differentiation ( Fig. 4a–c ). This lack of GM-CSF production by Bhlhe40 −/− T cells was also seen in T H 17 cultures that utilized TGF-β3 in place of TGF-β1 (ref. 26 ) ( Supplementary Fig. 7f ). Bhlhe40 −/− T H 1 and T H 17 cells showed increased IL-10 production relative to WT cells, while WT and Bhlhe40 −/− T H 2 cells showed similar, high-level IL-10 production ( Fig. 4a,b ). The increased IL-10 production in Bhlhe40 −/− T H 1 cells came largely from IFN-γ + cells, while in T H 17 cultures it came from both IL-17A + and IL-17A − populations ( Fig. 4d ). We further tested whether the increased IL-10 production by Bhlhe40 −/− T H cells could contribute to their diminished GM-CSF production. Co-culture of congenically marked WT and Bhlhe40 −/− T H cells under non-polarizing conditions showed that increased IL-10 secretion and decreased GM-CSF secretion were both cell-intrinsic properties of Bhlhe40 −/− T H cells ( Fig. 4e ). We tested whether abnormal GM-CSF and IL-10 production by Bhlhe40 −/− CD4 + T cells could be restored by the reintroduction of Bhlhe40. Retrovirally transduced Bhlhe40 −/− T H 1 and T H 17 cells overexpressing Bhlhe40 produced increased levels of GM-CSF and decreased levels of IL-10 compared with non-transduced Bhlhe40 −/− T cells or Bhlhe40 −/− T cells transduced by an empty retrovirus ( Supplementary Fig. 8 ). Overexpressing Bhlhe40 modestly increased GM-CSF and decreased IL-10 production by WT T H 17 cells, but had little effect on WT T H 1 cells. Molecular analysis of Bhlhe40-regulated target genes We performed expression microarray analysis on WT and Bhlhe40 −/− CD4 + T cells cultured in T H 1, T H 2 and T H 17 conditions and validated these results by quantitative RT-PCR for selected transcripts ( Fig. 5 ). This analysis confirmed that Bhlhe40 −/− T cells were able to acquire characteristics largely reflective of normal T H 1, T H 2 or T H 17 differentiation, including their expression of signature cytokines and transcription factors ( Fig. 5a,d ). However, a common set of genes was affected by the loss of Bhlhe40 across two or more T H lineages ( Fig. 5b,c and e ), including reduced expression of Csf2 , Il3 , Il1a , Ccl1 , Ifitm3 and Ptgs2 . Notably, expression levels of Il10 , Ikzf3 (Aiolos) and Xcl1 were increased in Bhlhe40 −/− T cells. We confirmed reduced secretion of IL-3 by Bhlhe40 −/− CD4 + T cells following stimulation with anti-CD3 alone or anti-CD3 and anti-CD28 ( Supplementary Fig. 7d ). 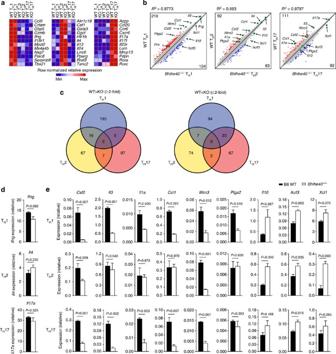Figure 5:Transcriptional analysis of Bhlhe40-deficient THcells. (a) Heat map of gene expression for selected TH1, TH2 and TH17 lineage-specific genes in polarized WT andBhlhe40−/−THcells. (b) Pairwise comparison of WT andBhlhe40−/−TH1, TH2 and TH17 cells. Probes that are overexpressed ≥2-fold in the indicated populations are shown in red or blue. Numbers in corners indicate the total number of probes meeting these conditions. Probes for selected relevant genes are shown in green. Coefficients of determination (R2) are indicated for each comparison. (c) Venn diagrams showing the overlap of probes differentially expressed by WT and KO THcell lineages. Numbers in regions indicate the number of probes with greater than or equal to a twofold difference in expression (WT>KO or WT<KO). (d) Quantitative RT-PCR analysis ofIfng,Il4andIl17aexpression in WT andBhlhe40−/−TH1, TH2 and TH17 cells (n=3 per group). (e) Quantitative RT-PCR analysis of the expression of the indicated nine genes in WT andBhlhe40−/−TH1, TH2 and TH17 cells (n=3 per group). Figure 5: Transcriptional analysis of Bhlhe40-deficient T H cells. ( a ) Heat map of gene expression for selected T H 1, T H 2 and T H 17 lineage-specific genes in polarized WT and Bhlhe40 −/− T H cells. ( b ) Pairwise comparison of WT and Bhlhe40 −/− T H 1, T H 2 and T H 17 cells. Probes that are overexpressed ≥2-fold in the indicated populations are shown in red or blue. Numbers in corners indicate the total number of probes meeting these conditions. Probes for selected relevant genes are shown in green. Coefficients of determination ( R 2 ) are indicated for each comparison. ( c ) Venn diagrams showing the overlap of probes differentially expressed by WT and KO T H cell lineages. Numbers in regions indicate the number of probes with greater than or equal to a twofold difference in expression (WT>KO or WT<KO). ( d ) Quantitative RT-PCR analysis of Ifng , Il4 and Il17a expression in WT and Bhlhe40 −/− T H 1, T H 2 and T H 17 cells ( n =3 per group). ( e ) Quantitative RT-PCR analysis of the expression of the indicated nine genes in WT and Bhlhe40 −/− T H 1, T H 2 and T H 17 cells ( n =3 per group). Full size image To examine whether the Il3 / Csf2 and Il10 loci were directly bound by Bhlhe40, we performed an analysis of Bhlhe40 ChIP-Seq data generated from CH12 cells by the Mouse Encyclopedia of DNA Elements (ENCODE) Consortium [44] . RNA sequencing (RNA-Seq) performed on this B-cell lymphoma line by the same Consortium showed these cells to express Bhlhe40 , Il3 , Csf2 and Il10 . Within the Il3 / Csf2 locus, Bhlhe40 bound multiple sites, including a previously identified distal enhancer located ~30 kb downstream of Csf2 that regulates the expression of both cytokine genes in this locus [45] ( Supplementary Fig. 9a ). Within the Il10 locus, Bhlhe40 also bound multiple sites, including two known regulatory elements [46] , [47] ( Supplementary Fig. 9b ). In both loci, many regions bound by Bhlhe40 were also bound by the general transcriptional regulators p300 (refs 48 , 49 ) and BRG1 (ref. 45 ) and the T H cell subset-specific transcription factors T-bet (ref. 50 ) and RORγt (ref. 49 ). Bhlhe40 is likely one of many transcriptional regulators present at these regions working in concert to control gene expression. IL-10R blockade renders Bhlhe40 −/− mice susceptible to EAE As our expression microarray experiments demonstrate that Bhlhe40 deficiency leads to the dysregulation of hundreds of genes in polarized T H cells, we expect that the summation of these changes in gene expression underlies the T cell-intrinsic requirement for Bhlhe40 in T-cell encephalitogenicity. Nevertheless, we sought to test whether the administration of exogenous GM-CSF could render Bhlhe40 −/− mice susceptible to EAE. In two individual experiments, Bhlhe40 −/− mice treated daily with either 10 or 100 ng per day recombinant murine GM-CSF intraperitoneally beginning on the day of immunization did not develop clinical EAE ( n =3–5 mice per experiment). In both of these experiments, control WT mice experienced a typical course of EAE, indicating successful immunization. Systemic GM-CSF treatment at a dose of 10 ng per day was reported to replace endogenous GM-CSF in Csf2 −/− mice, such that these mice developed EAE when GM-CSF was administered after immunization [51] . Therefore, we take our results to indicate that Bhlhe40 −/− mice resist EAE for reasons beyond just their defective production of GM-CSF by T cells. We also tested whether blockade of IL-10 signalling could affect the development of EAE in Bhlhe40 −/− mice. Groups of WT or Bhlhe40 −/− mice were treated biweekly with control rat IgG or anti-IL-10R blocking antibody, beginning 1 day prior to immunization and continuing throughout the course of the experiment. Anti-IL-10R antibody treatment of immunized WT mice led to the high incidence of early morbidity and a shock-like syndrome, characterized by ruffled fur, weight loss and a hunched posture, with rapid death prior to the onset of clinical EAE ( Fig. 6a ). This unexpected mortality, which we attribute to acute IL-10R blockade in the setting of a strong immune stimulus, was not apparent in immunized WT mice treated with control antibody, which experienced a typical course of EAE ( Fig. 6b and Table 1 ). Immunized Bhlhe40 −/− mice treated with anti-IL-10R antibody experienced only infrequent early morbidity. Those WT mice treated with anti-IL-10R antibody that did not succumb to an early death developed very severe EAE. Immunized Bhlhe40 −/− mice treated with control antibody resisted EAE, while nearly half of all Bhlhe40 −/− mice treated with anti-IL-10R antibody developed severe clinical EAE, like that of control antibody-treated WT mice. Overall, these results reveal that the pathogenicity of Bhlhe40 −/− autoreactive T cells is regulated by IL-10. 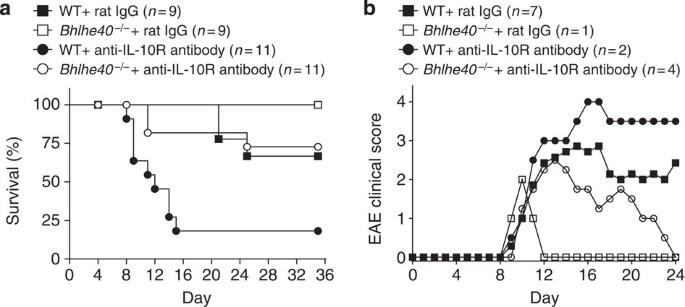Figure 6:IL-10R blockade rendersBhlhe40−/−mice susceptible to EAE. (a) Survival of WT orBhlhe40−/−mice after EAE induction and biweekly treatment with control rat IgG or anti-IL-10R antibody. Data are combined from three independent experiments. (b) Mean clinical scores of EAE in diseased WT orBhlhe40−/−mice treated biweekly with either control rat IgG or anti-IL-10R antibody. Data are combined from three independent experiments. Error bars are not shown for clarity. All s.e.m. values were ≤1. Figure 6: IL-10R blockade renders Bhlhe40 −/− mice susceptible to EAE. ( a ) Survival of WT or Bhlhe40 −/− mice after EAE induction and biweekly treatment with control rat IgG or anti-IL-10R antibody. Data are combined from three independent experiments. ( b ) Mean clinical scores of EAE in diseased WT or Bhlhe40 −/− mice treated biweekly with either control rat IgG or anti-IL-10R antibody. Data are combined from three independent experiments. Error bars are not shown for clarity. All s.e.m. values were ≤1. Full size image Table 1 Clinical EAE data in WT and Bhlhe40 −/− mice treated with rat IgG or anti-IL-10R antibody. Full size table Here we have shown that Bhlhe40 −/− mice are protected from immunization-induced autoimmune neuroinflammation. T H cells have a cell-intrinsic requirement for Bhlhe40 during encephalomyelitis, and in these cells Bhlhe40 transcriptionally regulates the production of GM-CSF and IL-10. In vivo blockade of IL-10R allows immunized Bhlhe40 −/− mice to develop EAE, indicating the important role of this cytokine in regulating autoreactive T-cell pathogenicity. Bhlhe40 −/− mice were also protected from adoptively transferred EAE using an encephalitogenic T H 1 cell line, but only when a low number of pathogenic T cells were transferred ( Supplementary Fig. 2e ). In this system, cytokine-producing host T H cells infiltrate the CNS and participate in regulating neuroinflammation [42] . Large numbers of adoptively transferred, autoreactive WT T H 1 cells were capable of overcoming a requirement for Bhlhe40 in host cells ( Supplementary Fig. 2f ). Overall, these results are reminiscent of experiments in which low numbers of an encephalitogenic T H 1 cell line were unable to induce disease in IL-17A-deficient mice, but in which higher cell numbers could initiate neuroinflammation [42] . We favour a model in which the explanation for our adoptive transfer results stems from a requirement for Bhlhe40 in host T H and γδ T cells, although it remains a possibility that Bhlhe40 also functions in non-T cells during adoptively transferred EAE. The characteristics that define pathogenic T H cells in EAE have been a subject of recent debate [24] , [25] , [26] . Neither IFN-γ nor IL-17, the signature cytokines of T H 1 and T H 17 cells, are required for the development of EAE [4] , [5] , yet in vitro derived T H 1 and T H 17 cells specific for myelin antigens both can induce encephalomyelitis [8] , [52] . These seemingly conflicting observations have been reconciled by the recent finding that GM-CSF, produced by both T H 1 and T H 17 cells, serves a non-redundant pro-inflammatory role in EAE development [8] , [9] , [10] , [11] , [12] . Control of Csf2 expression involves AP-1, NFAT, Runx1, NF-κB, histone acetylation and BRG1 recruitment [14] , [15] , [16] , [17] , [18] , [19] , [45] . c-Rel- and NF-κB1-deficient T cells produce less GM-CSF, but these factors may be non-selective in their impact on cytokine production [17] , [18] . Malt1, a protease regulating the NF-κB pathway, was reported to be required for GM-CSF production by T H 17 cells, but not T H 1 cells [53] , implying that the pathways that control GM-CSF production may not be the same in all T H cell lineages. In fact, we find that Bhlhe40 appears to play a less important role in regulating GM-CSF production in T H 2 cells compared with its role in T H 1 or T H 17 cells, as GM-CSF secretion is only partly abrogated in Bhlhe40 −/− T H 2 cells. Similarly, our observation that Bhlhe40 −/− mice can infrequently develop clinical EAE with some T-cell production of GM-CSF ( Supplementary Fig. 2a ) in the CNS indicates that Bhlhe40 is not absolutely required for Csf2 expression in T cells. Bhlhe41 (also known as Dec2, Sharp1 or Bhlhb3), the closest homologue to Bhlhe40, is expressed most highly in T H 2 cells among activated T H -cell subsets [40] , [54] , and perhaps this factor can substitute for Bhlhe40 in some settings in the regulation of Csf2 transcription. The role of RORγt in GM-CSF production by CD4 + T cells is controversial [10] , [11] , [12] . One study found that Rorc −/− CD4 + T cells activated in the presence of anti-IFN-γ- and anti-IL-12-neutralizing antibodies produced less GM-CSF than WT CD4 + T cells, but Rorc −/− T H 1 and T H 17 cells produced normal or even greater GM-CSF than WT T cells [10] . These investigators found that retroviral RORγt overexpression increased GM-CSF production, so despite these incongruous results, they suggested that RORγt drives GM-CSF production. A second study also showed that Rorc −/− T H 17 cells produced an increased amount of GM-CSF relative to WT T H 17 cells [11] , leading this group to suggest that RORγt is not required for GM-CSF production. We observed normal Rorc expression in Bhlhe40 −/− T H 17 cells in our microarrays ( Fig. 5a ), and speculate that Bhlhe40 directly regulates Csf2 expression. The recently described molecular signatures of pathogenic versus non-pathogenic T H 17 cells [26] includes four genes that we find to be selectively regulated by Bhlhe40 ( Csf2 and Il3 for pathogenic T H 17 cells; Il10 and Ikzf3 for non-pathogenic T H 17 cells) ( Fig. 5 ). Given these data, we believe that Bhlhe40 serves as a transcription factor that shapes the encephalitogenicity of T H 17 cells. Considering IL-10 production in particular, we find the largest difference between WT and Bhlhe40 −/− T H cells to be in T H 1 cultures or in cells from immunized mice cultured with IL-12. This type of IL-10 production by T H 1 cells has been reported to involve signals through ERK, STAT4 and c-Maf [33] . Our data point to a cell-intrinsic role for Bhlhe40 in regulating IL-10 production in T cells, and we speculate that Bhlhe40 serves as a direct negative regulator of Il10 . Bhlhe40 could be acting in T H cells in some cases as a transcriptional activator and in others as a transcriptional repressor on different direct target genes, perhaps based on its interactions with other transcription factors. Examples exist for both activating and repressive functions of Bhlhe40 (refs 55 , 56 ). It also remains possible that some genes whose expression is abnormal in Bhlhe40 −/− T H cells are indirect targets of Bhlhe40. Supporting the importance of IL-10 in EAE pathogenesis, we found that nearly half of all Bhlhe40 −/− mice treated with an anti-IL-10R blocking antibody developed EAE. Although IL-10-deficient mice are known to develop more severe EAE than WT mice [28] , [29] , [30] , they have not been reported to exhibit early mortality prior to the onset of encephalomyelitis. We speculate that the sudden inhibition of IL-10 signalling by anti-IL-10R antibody in our experiments is fundamentally different than the lifelong absence of this signalling, such that antibody-mediated blockade resulted in a pro-inflammatory cytokine-driven shock-like syndrome. Antibody-treated Bhlhe40 −/− mice were largely protected from this syndrome, implying that pro-inflammatory cytokines in these mice, perhaps including GM-CSF, were produced at lower levels. Interestingly, some Bhlhe40 −/− mice were fully protected from EAE even in the setting of IL-10R blockade, and we speculate that this was also due to their decreased levels of pro-inflammatory cytokines. Nevertheless, our results support the notion that Bhlhe40 −/− T H cells can be encephalitogenic in the setting of IL-10R blockade. Further experiments will be performed to determine whether Bhlhe40 −/− T H cells are themselves the critical source of IL-10 preventing autoimmunity in these mice. While we were preparing this manuscript, a separate study also identified Bhlhe40 as a transcription factor required for autoreactive CD4 + T-cell responses using the EAE system [57] . Martínez-Llordella et al. [57] identified Bhlhe40 as a gene whose expression was induced in activated CD4 + T cells in a CD28-dependent manner. These authors found Bhlhe40-deficient mice (a separately generated line than was used in our study [58] ) to be resistant to the induction of EAE, and found decreased CD4 + T cell production of several cytokines, including GM-CSF. Both our study and theirs found decreased IL-17A responses in immunized Bhlhe40 −/− mice, with both identifying this defect as cell-extrinsic based on immunization experiments in mixed bone marrow chimeras. Our in vitro experiments showing normal Il17a transcript and IL-17A production by Bhlhe40 −/− T H 17 cells also suggest no direct role for Bhlhe40 in controlling this cytokine. There are some key differences between our study and the work of Martínez-Llordella et al. [57] They observed MOG(35–55)-specific CD4 + T-cell responses in Bhlhe40 −/− mice to be only slightly reduced in frequency at day 7 after immunization as determined by tetramer staining, but to be completely absent when assessed with a proliferation assay or by ELISAs for IL-17A, IFN-γ and GM-CSF. In our assessment of CD4 + T-cell priming by ELISPOT assays using DLN cells at day 7 after immunization, we found essentially intact IL-2 and IFN-γ responses, partially decreased IL-17A responses and absent GM-CSF responses ( Fig. 3a,b ). We speculate that technical differences in the assay formats, cell culture densities or assay times could explain these discrepancies. An additional difference between our study and that of Martínez-Llordella et al. [57] is that we found normal IL-2 production after in vitro stimulation of Bhlhe40 −/− CD4 + T cells ( Supplementary Fig. 7a ), while they saw a ~50% reduction in IL-2 secretion. Our results are consistent with those of Miyazaki et al. [38] who reported normal IL-2 secretion by Bhlhe40 −/− CD4 + T cells, and we again speculate that differences in cell culture conditions may explain these discrepancies. Finally, our expression microarrays and phenotypic analysis of polarized Bhlhe40 −/− T H cells identified increased transcription and secretion of IL-10 by these cells compared with WT T H cells. Il10 was not identified as being differentially expressed in the transcriptional analysis performed by Martínez-Llordella et al. [57] , although we speculate that this may be related to their analysis of naive T cells activated under non-polarizing conditions at early time points (4 and 24 h). In conclusion, we have demonstrated that Bhlhe40 is required for the encephalitogenicity of CD4 + T cells, likely through its regulation of GM-CSF and IL-10 production. Bhlhe40 is also required for γδ T-cell production of GM-CSF. Bhlhe40 controls these cytokines transcriptionally, but further investigation will be required to understand the molecular details of this regulation. Moreover, the question of whether regulation of these cytokines by Bhlhe40 in T cells influences pathogenesis in other autoimmune or infectious diseases is intriguing. The role of GM-CSF in autoimmune disease has prompted clinical interest in therapeutics to target this cytokine in rheumatoid arthritis and multiple sclerosis [59] . Bhlhe40, or pathways that regulate its expression or function, could also represent therapeutic targets in human autoimmunity. Mice C57BL/6 (Taconic), B6.SJL (Taconic), B6.PL- Thy1 a /CyJ (Jackson), Rag1 −/− (on a C57BL/6 background, Jackson) and Bhlhe40 −/− mice [39] (backcrossed 10 generations to the C57BL/6 background) were maintained in our SPF facility. Experiments were performed with mice of either sex (groups were sex-matched within individual experiments) at 8–24 weeks of age. No Bhlhe40 −/− mice on the C57BL/6 background displayed lymphoproliferative disease in our colony throughout this age range, in keeping with a previous report of C57BL/6 Bhlhe40 −/− mice [38] . Flow cytometry of splenocytes and bone marrow from Bhlhe40 −/− mice in our colony at the ages used in these experiments showed normal leukocyte populations ( Supplementary Fig. 10 ). All animal experiments were approved by the Animal Studies Committee of Washington University. Bone marrow transplantation and T H cell transfers Bone marrow cells were collected from femurs and tibias of donor mice, and 10–20 million cells were injected intravenously into recipient mice following irradiation (1,200 rads). Mixed chimeras were prepared by mixing donor bone marrow cells at a 1:1 ratio before injection. Mice were used in experiments 13–16 weeks following transplantation. For cell transfers, total CD4 + T cells were magnetically purified from donor splenocytes (Invitrogen Dynabeads FlowComp Mouse CD4 kit, typical purity ~90–95%). CD4 + T cells (7 to 10 million) were injected intravenously into Rag1 −/− mice 1 day prior to the induction of EAE or immunization for the assessment of T-cell responses. Induction of EAE and immunizations For active EAE induction, mice were immunized subcutaneously with 100 μg MOG(35–55) (C S Bio Co.) emulsified in CFA (made with 5 mg ml − heat-killed Mycobacterium tuberculosis H37Ra (BD Difco) in incomplete Freund’s adjuvant (BD Difco)). Pertussis toxin (List Biological Laboratories) was injected intraperitoneally (300 ng) on days 0 and 2. Mice were observed for signs of EAE and graded on a standard 0–5 scale as described [11] . In some experiments, mice were treated daily with recombinant murine GM-CSF (Peprotech) at a dose of 10 ng per day or 100 ng per day intraperitoneally, beginning on the day of immunization and continuing throughout the course of the experiment. In some experiments, mice were treated with control rat IgG (Sigma) or anti-IL-10R monoclonal antibody (clone 1B1.3A, BioXcell) [60] . Mice were given 250 μg of antibody intraperitoneally two times per week, beginning 1 day prior to immunization. For histology experiments, spinal cords were dissected, fixed in formalin, embedded in paraffin, sectioned and stained with hematoxylin and eosin (H&E). For adoptively transferred EAE, MOG(35–55)-specific T H 1 cell lines were generated by culturing CD4 + T cells from MOG(35–55)-immunized CD90.1 congenic B6.PL- Thy1a /CyJ mice with MOG(35–55), irradiated C57BL/6 splenocytes, IL-2 and IL-12 for two or four rounds of stimulation [42] . Four days after the last stimulation, 5–10 million live T cells were intravenously transferred to recipient mice. For analysis of T-cell responses in DLNs, mice were immunized in hind footpads with 10 nanomoles MOG(35–55) or OVA(323–339) emulsified in CFA. Popliteal lymph nodes were collected on day 7. Cell preparation DLNs from immunized mice were digested with 250 μg ml −1 collagenase B (Roche) and 30 U ml −1 Dnase I (EMD) for 40–60 min at 37 °C with stirring in Iscove’s modified Dulbecco’s media containing 10% FCS, L -glutamine, sodium pyruvate, non-essential amino acids, penicillin/streptomycin and 2-mercaptoethanol (cIMDM). EDTA (5 mM final) was added and cells were incubated on ice for 5 min. Cells were passed through a 70-μm strainer before cell counting with trypan blue. Spleens were mashed between frosted glass slides and made into a single-cell suspension. Red blood cells were lysed with ACK lysis buffer. Cells were passed through a 70-μm strainer before cell counting with acetic acid. Brains and spinal cords were removed following perfusion with 30 ml PBS via cardiac puncture of the left ventricle. Organs were minced and digested with 500 μg ml −1 Type I collagenase (Sigma) and 10 μg ml −1 DNAse I (Sigma) in the presence of 0.1 μg ml −1 TLCK trypsin inhibitor (Sigma) and 10 mM Hepes (pH 7.4) in HBSS at room temperature for 1 h. Following centrifugation, cells were resuspended in 70% Percoll (Sigma) in HBSS and additional 37% and 30% layers were added above the cells. Gradients were centrifuged for 30 min at 1,200 g . The 30% Percoll layer containing debris was discarded, and the cells from the 37% layer were collected and washed in HBSS before stimulation or flow cytometry. Cell culture DLN cells from MOG(35–55)-immunized mice were cultured in cIMDM and stimulated with 10 μM MOG(35–55) for 4 days before supernatants were collected for ELISAs or before ICS. In some cases, IL-1β (10 ng ml −1 , BioLegend), IL-23 (20 ng ml −1 , BioLegend) or IL-12 (2 ng ml −1 , BioLegend) was added to the culture at set-up. Splenocytes or magnetically purified total splenic CD4 + T cells (Invitrogen Dynabeads FlowComp Mouse CD4 kit) from untreated mice cultured in cIMDM were stimulated with plate-bound anti-CD3 antibody (10 μg ml −1 , clone 145-2C11, BioLegend) with or without plate-bound anti-CD28 antibody for 48–72 h (5 μg ml −1 , clone 37.51, BioLegend). Supernatants were collected for ELISAs or ICS was performed on cells. In some experiments, splenocytes were cultured for 3 days with IL-1β and/or IL-23 without TCR stimulation. ICS was subsequently performed on these cells, gating on γδ T cells. For T H cell polarization, magnetically purified total CD4 + T cells (Invitrogen Dynabeads FlowComp Mouse CD4 kit) or naive CD4 + T cells (Stemcell Technologies Easysep Mouse Naive CD4 + T Cell Isolation kit, typical purity ~90–96%) were cultured in cIMDM with plate-bound anti-CD3 and anti-CD28 antibodies in the presence of cytokines (BioLegend except TGF-β3) and neutralizing antibodies (BioLegend except anti-IL-12) as follows. T H 1 conditions: IFN-γ (200 ng ml −1 ), IL-12 (2 ng ml −1 ), anti-IL-4 (5 μg ml −1 , clone 11B11). T H 2 conditions: IL-4 (10 ng ml −1 ), anti-IFN-γ (5 μg ml −1 , clone XMG1.2 or clone H22), anti-IL-12 (10 μg ml −1 , clone Tosh, a gift from Emil Unanue, Washington University). T H 17 conditions: TGF-β1 (2 ng ml −1 ) or TGF-β3 (2 ng ml −1 ) (Miltenyi), IL-6 (25 ng ml −1 ), IL-1β (10 ng ml −1 ), IL-23 (10 ng ml −1 ), anti-IL-4 and anti-IFN-γ. Cells were split at day 3, and on days 4–5 cells were either used for ICS or stimulated for 24 h with plate-bound anti-CD3 and anti-CD28 for assessment of cytokine secretion by ELISA. ELISPOT and ELISA assays ELISPOT assays were performed on Mutiscreen Filter Plates (Millipore). DLN cells from immunized mice were plated at 5 × 10 5 –1 × 10 6 cells per well in cIMDM and stimulated with 10 μM peptide or 1 μg ml −1 ConA overnight at 37°C. IL-2, IFN-γ and IL-10 ELISPOT antibody pairs were from BD Bioscience. IL-17 and GM-CSF ELISPOT antibody pairs and streptavidin-alkaline phosphatase were from BioLegend. Plates were developed with NBT/BCIP substrate (Roche) and spots were counted on an Immunospot counter (Cellular Technology Ltd.). ELISA assays were performed on Nunc Maxisorp plates using the same antibody pairs as above but were developed with streptavidin-HRP (BioLegend) and TMB substrate (BioLegend). Standard curves for these ELISAs were generated with purified cytokines. The Mouse IL-3 ELISA MAX kit was used to measure IL-3 (BioLegend). Flow cytometry All antibodies were used at a dilution of 1/200 except where noted. Streptavidin conjugates were used at a dilution of 1/400. The following anti-mouse antibodies were from BioLegend: FITC, APC or biotin anti-CD3e (145-2C11), PB anti-CD4 (RM4-5), APC-Cy7 or PerCP-Cy5.5 anti-CD8α (53-6.7), APC or biotin anti-TCR γδ (GL3), FITC anti-CD25 (PC61), PB anti-CD44 (IM7), FITC anti-B220 (RA3-6B2), FITC anti-CD45.1 (A20), APC or biotin anti-CD45.2 (104), PerCP-Cy5.5 anti-Siglec H (551), FITC anti-Ly6C (HK1.4), PE anti-Ly6G (1A8), PE-Cy7 anti-CD11b (M1/70), APC-Cy7 anti-CD11c (N418), PB anti-I-A/I-E (M5/114.15.2, used at 1/500), PE-Cy7 anti-IFN-γ (XMG1.2), PerCP-Cy5.5 anti-IL-17A (TC11-18H10.1), PE anti-GM-CSF (MP1-22E9), PE anti-KLH (RTK2758, isotype rat IgG2a, κ), APC or biotin anti-IL-10 (JES5-16E3) and streptavidin-APC. The following anti-mouse antibodies were from BD Biosciences: V450 anti-CD4 (RM4-5) and V500 anti-B220 (RA3-6B2). APC anti-CD62L (MEL-14), PE anti-CD25 (PC61.5), APC-e780 anti-CD45 (30-F11, used at 1/600), PE anti-Foxp3 (FJK-16s), eFluor660 anti-T-bet (eBio4B10), PerCP-eFluor710 anti-Gata-3 (TWAJ), APC anti-RORγt (AFKJS-9) and streptavidin-APC-e780 were from eBioscience. For ICS, cells were stimulated with PMA (50 ng ml −1 , Enzo Life Sciences) and ionomycin (1 nM, Enzo Life Sciences) in the presence of brefeldin A (1 μg ml −1 , Enzo Life Sciences) for 4–5 hours. Surface staining was performed in FACS buffer (0.5% BSA, 2 mM EDTA, 0.02% sodium azide in PBS) in the presence of Fc receptor blocking antibody (clone 93, BioLegend) for 20 min at 4 °C followed by streptavidin staining if necessary. Cells were fixed in 4% paraformaldehyde (Electron Microscopy Sciences) for 20 min at room temperature followed by permeabilization (0.1% BSA, 0.5% saponin in PBS) or with the BD Cytofix/Cytoperm Fixation and Permeabilization Kit. Cytokine staining was performed in permeabilization buffer for 20 min at 4 °C. Staining for intracellular Foxp3, T-bet, Gata-3 and RORγt was performed in the Foxp3/Transcription Factor Staining Buffer Set (eBioscience). Flow cytometry was performed on a FACSCanto II (BD Bioscience) and data was analysed with FlowJo (Tree Star Inc.). For microarray experiments, naive CD4 + T cells (CD4 + B220 − CD25 − CD44 lo CD62L hi ) were purified (98% purity) by cell sorting on a FACSAria II (BD Biosciences) after B-cell depletion using anti-B220 magnetic beads (Invitrogen). Expression microarrays Naive CD4 + T cells were cultured in T H 0, T H 1, T H 2 or T H 17 conditions for 4 days and stimulated for 4 h with PMA and ionomycin before total RNA was isolated (EZNA MicroElute Total RNA Kit, Omega Bio-Tek). RNA was amplified (Ovation PicoSL WTA System V2, Nugen), labelled (Encore Biotin Module, Nugen), fragmented and hybridized to Affymetrix Gene 1.0ST arrays. Array data were imported into Arraystar 5 software (DNAstar) and then normalized using the robust multi-array analysis method with quantile normalization. Probesets were curated according to a validated gene annotation, and only these probesets were utilized in subsequent analyses. Correlation analysis was performed using Arraystar 5. Heat maps were generated using GENE-E software (Broad Institute, http://www.broadinstitute.org/cancer/software/GENE-E/ ). For analysis of GSE14308 (ref. 61 ), which was performed on Affymetrix Mouse Genome 430 2.0 arrays, we also used the robust multi-array analysis method with quantile normalization using Arraystar 5 software. Quantitative RT-PCR Magnetically purified total splenic CD4 + T cells (Invitrogen Dynabeads FlowComp Mouse CD4 kit) were cultured in T H 1, T H 2 or T H 17 conditions for 4 days and stimulated for 4 h with plate-bound anti-CD3 and anti-CD28 before total RNA was isolated (EZNA MicroElute Total RNA Kit, Omega Bio-Tek). cDNA was synthesized (High Capacity RNA-to-cDNA Kit, Invitrogen) and quantitative real-time PCR was performed according to the manufacturer’s instructions with Power SYBR Green PCR Master Mix (Applied Biosystems) on a StepOnePlus Real-Time PCR system (Applied Biosystems). Expression of genes was determined relative to Hprt by the ΔC T method. The following primers were used for quantitative RT-PCR. Ccl1 , forward 5′-GGCTGCCGTGTGGATACAG-3′, reverse 5′-AGGTGATTTTGAACCCACGTTT-3′; Csf2 , forward 5′-GCCATCAAAGAAGCCCTGAA-3′, reverse 5′-GCGGGTCTGCACACATGTTA-3′; Hprt , forward 5′-TCAGTCAACGGGGGACATAAA-3′, reverse 5′-GGGGCTGTACTGCTTAACCAG-3′; Ifitm3 , forward 5′-CCCCCAAACTACGAAAGAATCA-3′, reverse 5′- ACCATCTTCCGATCCCTAGAC-3′; Ifng , forward 5′-GGATGCATTCATGAGTATTGC-3′, reverse 5′-CCTTTTCCGCTTCCTGAGG-3′; Ikzf3 , forward 5′-CTGAATGACTACAGCTTGCCC-3′, reverse 5′-GCTCCGGCTTCATAATGTTCT-3′; Il1a , forward 5′- CGAAGACTACAGTTCTGCCATT-3′, reverse 5′-GACGTTTCAGAGGTTCTCAGAG-3′; Il3 , forward 5′-GGGATACCCACCGTTTAACCA-3′, reverse 5′-AGGTTTACTCTCCGAAAGCTCTT-3′; Il4 , forward 5′-ATCATCGGCATTTTGAACGAGG-3′, reverse 5′- TGCAGCTCCATGAGAACACTA-3′; Il10 , forward 5′-AGCCTTATCGGAAATGATCCAGT-3′, reverse 5′-GGCCTTGTAGACACCTTGGT-3′; Il17a , forward 5′-TTTAACTCCCTTGGCGCAAAA-3′, reverse 5′-CTTTCCCTCCGCATTGACAC-3′; Ptgs2 , forward 5′-TGCACTATGGTTACAAAAGCTGG-3′, reverse 5′-TCAGGAAGCTCCTTATTTCCCTT-3′; Xcl1 , forward 5′-TAGCTGTGTGAACTTACAAACCC-3′, reverse 5′-ACAGTCTTGATCGCTGCTTTC-3′. ChIP-Seq data analysis Bhlhe40 ChIP-Seq data and RNA-Seq data performed by ENCODE/Stanford/Yale using CH12 cells were directly viewed in the University of California Santa Cruz (UCSC) Genome Browser on the NCBI37/mm9 mouse genome assembly. Discriminative DNA Motif Discovery (DREME) software (ref. 62 ) was used as part of the online version of MEME-ChIP ( http://meme.nbcr.net/meme/cgi-bin/meme-chip.cgi ) [63] to validate that Bhlhe40 ChIP-Seq data identified the expected consensus motif for Bhlhe40 (CACGTG) [64] with a significant E -value (4.8 × 10 −1,391 ). Raw data for the following ChIP-Seq data sets were downloaded from the Gene Expression Omnibus of the NCBI: GSE40463 (p300 in T H 1 and T H 2 cells) [48] , GSE33802 (T-bet in T H 1 cells) [50] , GSE20898 (Gata-3 in T H 2 cells) [65] , GSE40918 (RORγt and p300 in T H 17 cells) [49] and GSE23719 (BRG1 in stimulated T H 1, T H 2, and T H 17 cells) [66] . Each of these data sets was put through the following pipeline of analysis within Galaxy ( http://usegalaxy.org/ ) [67] , [68] , [69] : FASTQ files were groomed, mapped to the NCBI37/mm9 mouse genome assembly using Bowtie, converted from SAM to BAM files and peak called using MACS software. Tracks were then viewed in the UCSC Genome Browser. Cloning of Bhlhe40 and retroviral transduction The murine Bhlhe40 full-length cDNA (coding for amino acids 2–411) was cloned with the addition of 5′ and 3′ BglII sites, and a Kozak sequence upstream of an N-terminal Myc tag from cDNA derived from GM-CSF-derived bone marrow dendritic cells. The following primers were used: forward, 5′-AATAAGATCTCCACCATGGCAGAACAGAAGCTCATTTCTGAAGAAGACTTGAACGAACGGA TCCCCAGCGC-3′, reverse, 5′-ATAAAGATCTCCCTCCAGAGTTTAGTCTTTGGTTTCT-3′. The resulting fragment was digested with BglII and cloned into the BglII site of the GFP-RV vector which contains an internal ribosome entry sequence upstream of GFP [70] . Retroviral vectors were transfected into Phoenix E cells by calcium phosphate coprecipitation [70] , and viral supernatants were collected after 2 days of culture. Magnetically purified total CD4 + T cells (Invitrogen Dynabeads FlowComp Mouse CD4 kit) were stimulated in T H 1 or T H 17 conditions, and viral supernatants were used to infect T cells by spin infection at 2,000 r.p.m. in the presence of 2 μg ml −1 polybrene for 1 h on day 1 after activation. Cells were used for intracellular flow cytometry on day 4 of culture. Statistical analysis Differences between groups were analysed by an unpaired, two-tailed Student’s t -test (Prism; GraphPad Software, Inc.), with P ≤0.05 considered significant. Accession codes: Microarray data sets have been deposited in GEO Data sets under accession code GSE49166 . How to cite this article: Lin, C.-C. et al. Bhlhe40 controls cytokine production by T cells and is essential for pathogenicity in autoimmune neuroinflammation. Nat. Commun. 5:3551 doi: 10.1038/ncomms4551 (2014).